The unusual dynamics of parasite actin result from isodesmic polymerization Previous reports have indicated that parasite actins are short and inherently unstable, despite being required for motility. Here we re-examine the polymerization properties of actin in Toxoplasma gondii , unexpectedly finding that it exhibits isodesmic polymerization in contrast to the conventional nucleation–elongation process of all previously studied actins from both eukaryotes and bacteria. Polymerization kinetics of actin in T. gondii lacks both a lag phase and critical concentration, normally characteristic of actins. Unique among actins, the kinetics of assembly can be fit with a single set of rate constants for all subunit interactions, without need for separate nucleation and elongation rates. This isodesmic model accurately predicts the assembly, disassembly and the size distribution of actin filaments in T. gondii in vitro , providing a mechanistic explanation for actin dynamics in vivo . Our findings expand the repertoire of mechanisms by which actin polymerization is governed and offer clues about the evolution of self-assembling, stabilized protein polymers. Actin shares a common fold with a superfamily of proteins that includes sugar kinases, Hsp70, and actin-related proteins, including bacterial homologues of actin (that is, MreB, ParM and so on) [1] . Among this group, actins characteristically cycle between monomeric and filamentous forms using a nucleation–elongation mechanism for polymerization, which supports structure, mechanics and motility in cells [2] . Apicomplexan parasites, such as Toxoplasma and Plasmodium , are ancient, divergent eukaryotes that also require actin polymerization for motility [3] , [4] and active invasion of host cells [5] . Despite this requirement, the vast majority of parasite actin remains unpolymerized in vivo [6] , [7] and purified parasite actins form very short filaments in vitro [8] , [9] , [10] . Actin in T. gondii (TgACTI) is only ~80% identical to mammalian or yeast actin (ScACT) [6] and differences in the molecular interactions responsible for inter-strand filament contacts contribute to the instability of parasite actins [11] . It has remained enigmatic how the seemingly inefficient polymerization and transient nature of actin filaments support motility in these organisms. Conventional actins, as well as the actin-related protein Arp1, undergo cooperative assembly to polymerize head-to-tail into two inter-twined helical strands that form a filament [12] . Polymerization occurs by a nucleation–elongation mechanism in which filaments elongate rapidly from nuclei that assemble slowly and only if the actin concentration exceeds a characteristic critical concentration (Cc) [13] . Polymerization from monomeric subunits displays a slow nucleation step because of the instability of dimer and trimer intermediates, resulting in a lag phase in the time course of polymerization [14] . In contrast to a nucleation–elongation mechanism, protein polymers can theoretically assemble by an isodesmic mechanism, which is non-cooperative and does not require a nucleus to initiate polymerization [15] , [16] . During isodesmic polymerization, all monomer–polymer interactions occur with equal affinity and the amounts of both monomer and polymer increase with total protein concentration, in contrast to cooperative assembly, where the monomer concentration plateaus upon reaching the Cc [15] . All well-studied actins, from yeast, amoeba and animal cells [12] , as well as from bacterial actin-like homologues [17] , display nucleation–elongation polymerization, which is generally regarded as a conserved property of actins. Given the unusual nature of parasite actins, we challenged the assumption that a standard nucleation–elongation mechanism could account for actin polymerization in more distant eukaryotic species such as T. gondii . Our findings indicate that TgACTI actin assembles by a process that is largely isodesmic, thus revealing a novel means of assembly for a cytoskeletal protein polymer. These findings have implications for the regulation of assembly and turnover of filaments that help explain the unusual actin dynamics observed in vivo . TgACTI exhibits unusual polymerization kinetics We began by re-examining the polymerization of TgACTI by light scattering, using recombinant protein purified from baculovirus as described previously [11] . Polymerization was very limited at low protein concentrations but increased steadily over time at higher concentrations ( Fig. 1a ). Notably, the time course displayed no lag in the initiation of TgACTI polymerization at any of the concentrations tested ( Fig. 1a ). A previous study of the polymerization kinetics of TgACTI, as determined by tryptophan quenching, reported a lag phase but only at very low concentrations of protein [8] . Indeed, a lag phase is not exclusive to a nucleation–elongation mechanism, because this feature can also be observed for an isodesmic process when k off > k on [18] . When we examined the initial time of polymerization by light scattering over a wide range of concentrations, no lag phase was present ( Fig. 1a , right). Instead, the rate of polymerization increased in proportion to the concentration of protein, and continued to rise over the 2-h time frame ( Fig. 1a ). In contrast, actin from Saccharomyces cerevisiae , ScACT, expressed in baculovirus and purified in parallel, showed the typical lag, elongation and plateau phases characteristic of conventional actins ( Fig. 1b ; refs 13 , 14 ). 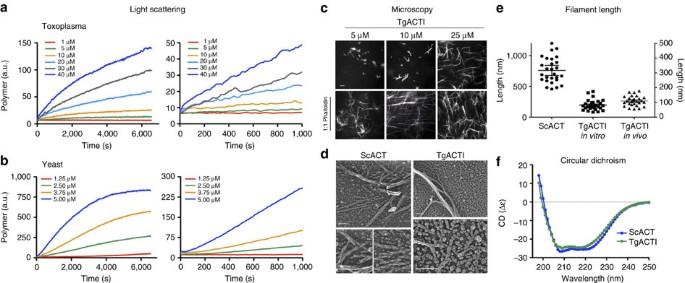Figure 1: Concentration-dependent polymerization of TgACTI versus ScACT. (a) Light scattering (arbitrary units, a.u.) versus concentrations (μM) of TgACTI. Plot at right shows the initial time course expanded to highlight the lack of lag phase. (b) Light scattering (arbitrary units, a.u.) versus concentrations (μM) of ScACT. Initial plots show evidence of lag (expanded plot at right) and plateau at later time points. (c) Fluorescence microscopy of polymerized TgACTI visualized with 0.33 μM Alexa 488-phalloidin±equimolar amounts of unlabelled Ph (1:1). Scale bar, 5 μM. (d) Quick-freeze, deep-etch electron micrographs of ScACT (5 μM) versus TgACTI (40 μM) polymerized in F-buffer. Scale bars, 100 nm. (e) Lengths of actin filaments measuredin vitrofor ScACT and TgACTI as ind, or for TgACTIin vivoas reported previously8. Leftyaxis, ScACT; rightyaxis, TgACTI. Means±s.d. (f) Circular dichroism measurements of purified ScACT versus TgACTI, 0.4 μM. All panels are representative experiments of three or more similar experiments. Figure 1: Concentration-dependent polymerization of TgACTI versus ScACT. ( a ) Light scattering (arbitrary units, a.u.) versus concentrations (μM) of TgACTI. Plot at right shows the initial time course expanded to highlight the lack of lag phase. ( b ) Light scattering (arbitrary units, a.u.) versus concentrations (μM) of ScACT. Initial plots show evidence of lag (expanded plot at right) and plateau at later time points. ( c ) Fluorescence microscopy of polymerized TgACTI visualized with 0.33 μM Alexa 488-phalloidin±equimolar amounts of unlabelled Ph (1:1). Scale bar, 5 μM. ( d ) Quick-freeze, deep-etch electron micrographs of ScACT (5 μM) versus TgACTI (40 μM) polymerized in F-buffer. Scale bars, 100 nm. ( e ) Lengths of actin filaments measured in vitro for ScACT and TgACTI as in d , or for TgACTI in vivo as reported previously [8] . Left y axis, ScACT; right y axis, TgACTI. Means±s.d. ( f ) Circular dichroism measurements of purified ScACT versus TgACTI, 0.4 μM. All panels are representative experiments of three or more similar experiments. Full size image The differences between yeast and TgACTI polymerization were apparent, despite the fact that light scattering is not directly proportional to filament mass because the light-scattering signal is also influenced by bundling. With some other methods, such as fluorescence of pyrene–actin, the signal is proportional only to filament mass [19] . In the pyrene–actin method, actin is labelled with pyrene on a conserved cysteine residue. TgACTI has this conserved cysteine (Cys375), and we were able to label Cys375 with pyrene. However, we found that pyrene–TgACTI did not show enhanced fluorescence when polymerization was induced (C. Ma, unpublished). Although the effects of bundling on the signal meant that we were not able to directly model the assembly kinetics from the light-scattering traces, dramatic differences were evident between the traditional nucleation–elongation process exhibited by ScACT and the unconventional process exhibited by TgACTI. Although TgACTI showed evidence of polymerization by light scattering, it did not form conventional length filaments detectable by fluorescence phalloidin (Ph) staining unless incubated with equimolar concentrations of Ph (that is, at 5 μM; Fig. 1c ), consistent with previous reports [11] . This requirement was overcome at higher protein concentrations (that is, 25–40 μM), allowing visualization of bundles of long filaments that were detected by adding trace amounts of labelled Ph and fluorescence microscopy ( Fig. 1c ). When a high concentration of TgACTI was polymerized in F-buffer and examined by quick-freeze, deep-etch electron microscopy (EM), occasional filament bundles were surrounded by many small heterogeneously sized oligomers and short filaments ranging from 25 to 100 nm, which are similar to previous in vivo measurements [8] ( Fig. 1d,e ). In contrast, ScACT formed much longer filaments (that is, 500–1,500 nm) with a typical right-handed helical pattern of two protofilaments, which also occasionally formed bundles ( Fig. 1d,e ). The short filaments formed by TgACTI had a conventional double-stranded structure but showed less evidence of a helical pattern when compared with ScACT ( Fig. 1d ). The failure of TgACTI to form filaments at lower concentrations was not because of a general defect in folding because circular dichroism measurements indicated a similar secondary structure compared with that of ScACT ( Fig. 1f ). Inefficient sedimentation of heterogeneous TgACTI filaments When conventional actins undergo polymerization, nearly all of the polymer assumes the form of long filaments that sediment efficiently at 100,000 g (ref. 20 ). Previous studies using low concentrations (that is, below 5 μM) of TgACTI have reported that sedimentation requires higher g forces than conventional actins (that is, 350,000 g for 1 h; ref. 8 ). Given our findings for concentration dependence of TgACTI polymerization above, we examined the influence of protein concentration on the efficiency of sedimentation. When 5 μM TgACTI was polymerized in F-buffer and centrifuged at 100,000 g , ~30% of the protein appeared in the pellet ( Fig. 2a , top). Addition of Ph at an equimolar ratio caused a greater fraction of TgACTI to shift to the pellet (~60%; Fig. 2a , top). In contrast, centrifugation at 350,000 g was sufficient to pellet the majority of TgACTI, both in the presence and absence of Ph (~85–90%; Fig. 2a , top). At higher protein concentrations (that is, 30 μM), ~37% of TgACTI pelleted on centrifugation at 100,000 g ( Fig. 2a , middle). Addition of Ph and centrifugation at 100,000 g , or centrifugation at 350,000 g , was sufficient to sediment nearly all of the TgACTI (~90%; Fig. 2a , middle). In comparison, >90% of ScACT, expressed and purified in the same manner as TgACTI, was found in the pellet after incubation in F-buffer, regardless of the centrifugation speed or the presence of Ph ( Fig. 2a , bottom). These findings indicate that although TgACTI undergoes dose-dependent polymerization, it forms oligomers that sediment far less efficiently than conventional actins. 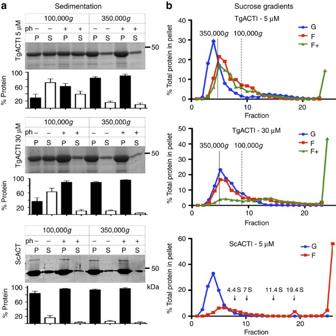Figure 2: TgACTI forms small heterogeneous polymers. (a) TgACTI (5 μM top versus 30 μM middle) was polymerized in F-buffer for 1 h at room temperature±equimolar Ph and centrifuged at 100,000 or 350,000gfor 1 h at room temperature. Pellet (P) or precipitated supernatant (S) fractions were resolved on a 12% SDS–polyacrylamide gel, stained with SYPRO-Ruby and quantified by phosphorimager analysis. ScACT (5 μM, bottom) was analysed in parallel. Mean±s.d.,n=3 or more experiments combined in graphs; representative gels are shown. (b) Sedimentation of TgACTI (5 μM top, 30 μM middle) in G-buffer (G, blue), F-buffer (F, red) or F-buffer with equimolar Ph (F+, green) by sucrose density centrifugation. ScACT (5 μM) was analysed in a parallel gradient. Dashed and solid black lines correspond to the proportion of TgACTI that would be found in the 100,000 and 350,000gpellets under standard sedimentation conditions as ina. Size standards are denoted with black arrows. All panels are representative of three or more similar experiments. Figure 2: TgACTI forms small heterogeneous polymers. ( a ) TgACTI (5 μM top versus 30 μM middle) was polymerized in F-buffer for 1 h at room temperature±equimolar Ph and centrifuged at 100,000 or 350,000 g for 1 h at room temperature. Pellet (P) or precipitated supernatant (S) fractions were resolved on a 12% SDS–polyacrylamide gel, stained with SYPRO-Ruby and quantified by phosphorimager analysis. ScACT (5 μM, bottom) was analysed in parallel. Mean±s.d., n =3 or more experiments combined in graphs; representative gels are shown. ( b ) Sedimentation of TgACTI (5 μM top, 30 μM middle) in G-buffer (G, blue), F-buffer (F, red) or F-buffer with equimolar Ph (F+, green) by sucrose density centrifugation. ScACT (5 μM) was analysed in a parallel gradient. Dashed and solid black lines correspond to the proportion of TgACTI that would be found in the 100,000 and 350,000 g pellets under standard sedimentation conditions as in a . Size standards are denoted with black arrows. All panels are representative of three or more similar experiments. Full size image To evaluate the size distribution of polymerized TgACTI, samples were subjected to density gradient centrifugation. When 5 μM TgACTI incubated in non-polymerizing G-buffer was analysed by sucrose gradient sedimentation, the majority of protein was found near the top of the gradient ( Fig. 2b , top). At higher protein concentrations (that is, 30 μM) in G-buffer, TgACTI sedimented more rapidly, appearing farther down the gradient ( Fig. 2b , middle). Incubation of 5 or 30 μM TgACTI in polymerizing F-buffer shifted the protein distribution further down the gradient, although the majority of protein was still found in lighter fractions under both conditions ( Fig. 2b ). Following the addition of Ph, ~15% of the 5 μM actin was shifted to the pellet, whereas the majority of 30 μM actin sedimented into the pellet ( Fig. 2b ). In contrast to the heterogeneous behaviour of TgACTI, sucrose gradient sedimentation of ScACT produced two discrete populations at opposite ends of the gradient. In G-buffer, the majority of ScACT was found in light fractions (S<4.4 standard for BSA), likely corresponding to monomers and a mixture of dimers ( Fig. 2b , bottom). However, in F-buffer, the majority of ScACT was found in the pellet, consistent with polymerization into long filaments ( Fig. 2b , bottom). To estimate the size of TgACTI polymers, we estimated the proportion of actin found in the pellet after F-buffer incubation and high-speed centrifugation at 100,000 or 350,000 g (data from Fig. 2a ). These estimated amounts of pelleted actin were plotted against the cumulative fractions of the sucrose gradients ( Fig. 2b , dashed line, solid line, respectively) to estimate the relative size of the filaments. From this comparison, it was evident that TgACTI filaments are not long, like those of yeast, which sediment rapidly. In contrast, TgACTI filaments are much shorter, and their length distribution is more heterogeneous. To provide a better estimate of the sizes of actin oligomers formed by TgACTI, we examined protein samples by dynamic light scattering and used an autocorrelation function to estimate hydrodynamic radius (Rh), mass and polydispersity. ScACT suspended in G-buffer was detected primarily as a single peak, with a Rh of 3.6 nm and approximate mass of 67 kDa ( Table 1 ). This size estimate possibly represents an average of monomer (estimated Rh 3.0) (ref. 21 ) and dimer forms (estimated Rh 3.8–4.1 for low-pitch and high-pitch dimer, respectively, as estimated using Stokes–Einstein theory). Addition of F-buffer to ScACT shifted the size to the upper end of the spectrum that was detectable by the instrument (that is, >10 9 kDa), consistent with assembly of actin into long polymers ( Table 1 ). The behaviour of TgACTI in G-buffer indicated a much larger average Rh and mass than that predicted for monomer, consistent with a range of small oligomers from 2 to 5 subunits at 1 μM that shifted to 5–10 subunits at 5 μM ( Table 1 , Supplementary Table S1 ). Addition of F-buffer shifted the size of TgACTI to an intermediate range with an average size of ~7,000 kDa, and a much broader polydispersity, consistent with a variety of oligomers from 35 to 500 subunits but without the extremely large polymers seen in ScACT ( Table 1 , Supplementary Table S1 ). The estimated size of TgACTI oligomers formed in G-buffer is consistent with globular aggregates previously reported by EM [8] , [11] , and the size distribution in F-buffer corresponds to observations of filaments observed by EM above, and reported previously [8] , [11] . The length distribution of TgACTI filaments depended on the concentration of TgACTI in a continuous manner, with longer filaments at higher concentrations of protein. In contrast, the length distribution of ScACT filaments displayed an abrupt transition to a population of long filaments when the protein concentration exceeded the Cc ( Fig. 1d , Table 1 , Supplementary Table S1 ). These different behaviours of filament length with respect to protein concentrations are consistent with predictions based on isodesmic versus nucleation–elongation modes of assembly. Table 1 Dynamic light scattering of actins in solution. Full size table TgACTI polymerizes by an isodesmic process Having established that TgACTI polymerizes more robustly at higher concentrations than those used in previous analyses, we revisited the question of the existence of a Cc. We examined the amount of protein in the supernatant and pellet after incubation for 1 h at room temperature in F-buffer (pH 8.0) and centrifugation for 1 h at 100,000 g . If TgACTI underwent nucleation–elongation polymerization similar to conventional actins, the concentration of protein in the supernatant would be expected to plateau at the Cc [13] , [14] . Strikingly, this was not observed. Rather, the amount of protein in the supernatant continued to increase up to 100 μM TgACTI, the highest concentration tested ( Fig. 3a ). The absence of a clear plateau in the supernatant was also observed when TgACTI was polymerized in KMEI buffer (pH 7.2; Fig. 3b ), indicating that this behaviour is not attributed to some unusual salt or pH preference. In contrast, polymerization of ScACT under similar conditions showed a marked plateau in the concentration of the supernatant and a clear Cc below which polymer was not detected ( Fig. 3c ). Purified TgACTI was also polymerized for 20 h, and the steady-state levels of polymerization were measured by light scattering, as described previously [11] . The amount of polymerized TgACTI increased proportionally to the total amount used in the reaction, and these data were fit using a linear or quadratic equation ( Fig. 3d ). The intercept of this curve crosses the x axis at very low concentration, but there was no range where polymerization did not occur ( Fig. 3d inset). When TgACTI polymerization reactions were allowed to go to steady state (that is, >20 h) and separated by sedimentation, again there was no obvious Cc, although above 10 μM, the majority of TgACTI was found in the pellet ( Fig. 3e ). Collectively, these results are inconsistent with a fixed Cc typical of a nucleation–elongation mechanism, but instead are explained by an isodesmic mechanism of polymerization. 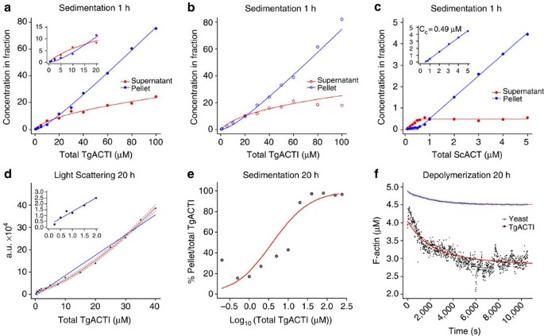Figure 3: TgACTI polymerizes by an isodesmic process. (a) Polymerization of TgACTI in F-buffer (pH 8.0) for 1 h followed by centrifugation at 100,000gfor 1 h at room temperature. The points are experimental results for the concentration of protein in the pellet (blue) or supernatant (red), plotted versus initial total concentration. The solid-line curves are the results of simulations using the isodesmic model. Inset shows the concentration range from 0.5 to 20 μM. (b) Similar sedimentation analysis performed as inaexcept KMEI (see Methods section; pH 7.2). (c) Polymerization of ScACT in F-buffer (pH 8.0) for 1 h followed by centrifugation at 100,000gfor 1 h at room temperature. Inset shows linear regression plot of lower concentrations (0.5–5 μM) used to estimate the Cc. (d) Polymerization of TgACTI in F-buffer at steady state (that is, 20 h), as monitored by light scattering. Linear regression (blue) or non-linear (red) fit curves are shown. Dotted line indicates 95% confidence interval. Mean, n≥3 experiments. Lower concentrations are expanded in inset. (e) Sedimentation of TgACTI polymerized to steady state in F-buffer for 20 h. Centrifugation at 100,000gfor 1 h at room temperature. The points are experimental data, and the solid curve is the result of a simulation with the isodesmic model. (f) Dilution-induced depolymerization of TgACTI versus ScACT. Steady-state samples polymerized for 20 h were diluted fourfold in F-buffer, and depolymerization was monitored by light scattering. The red curve is the prediction from the isodesmic model for TgACTI and from a nucleation–elongation model for ScACT. Unless otherwise noted, all panels are representative experiments of three or more similar experiments. Figure 3: TgACTI polymerizes by an isodesmic process. ( a ) Polymerization of TgACTI in F-buffer (pH 8.0) for 1 h followed by centrifugation at 100,000 g for 1 h at room temperature. The points are experimental results for the concentration of protein in the pellet (blue) or supernatant (red), plotted versus initial total concentration. The solid-line curves are the results of simulations using the isodesmic model. Inset shows the concentration range from 0.5 to 20 μM. ( b ) Similar sedimentation analysis performed as in a except KMEI (see Methods section; pH 7.2). ( c ) Polymerization of ScACT in F-buffer (pH 8.0) for 1 h followed by centrifugation at 100,000 g for 1 h at room temperature. Inset shows linear regression plot of lower concentrations (0.5–5 μM) used to estimate the Cc. ( d ) Polymerization of TgACTI in F-buffer at steady state (that is, 20 h), as monitored by light scattering. Linear regression (blue) or non-linear (red) fit curves are shown. Dotted line indicates 95% confidence interval. Mean, n≥3 experiments. Lower concentrations are expanded in inset. ( e ) Sedimentation of TgACTI polymerized to steady state in F-buffer for 20 h. Centrifugation at 100,000 g for 1 h at room temperature. The points are experimental data, and the solid curve is the result of a simulation with the isodesmic model. ( f ) Dilution-induced depolymerization of TgACTI versus ScACT. Steady-state samples polymerized for 20 h were diluted fourfold in F-buffer, and depolymerization was monitored by light scattering. The red curve is the prediction from the isodesmic model for TgACTI and from a nucleation–elongation model for ScACT. Unless otherwise noted, all panels are representative experiments of three or more similar experiments. Full size image We modelled the polymerization kinetics of TgACTI based on sedimentation assays using either conventional nucleation–elongation mechanism, as described previously [22] , or an isodesmic interaction, where the association and dissociation rate constants were assumed to be the same for each step in the polymerization reaction ( Fig. 4a ). Surprisingly, the isodesmic model does an excellent job of describing the extent of polymerization over the full range of actin concentrations ( Fig. 4b ). The isodesmic model predicts rate constants of k on =5.9 × 10 −5 μM −1 s −1 and k off =4.0 × 10 −4 s −1 , both remarkably low in comparison with the rate constants for elongation of conventional actin, for which the on-rate constant is typically ~10 μM −1 s −1 (refs 12 , 22 ). The rate constants for TgACTI give a binding affinity of 6.8 μM, consistent with the observed low rate of TgACTI polymerization at low concentrations and increased abundance of filaments with increasing concentration. Simulation of the polymerization kinetics using the isodesmic model generated curves that closely matched the proportion of TgACTI in the supernatant versus pellet at both 1 and 20 h (curves in Fig. 3a,e ). Structural modelling and molecular dynamics support a role for an isodesmic mechanism in explaining the behaviour of TgACTI. Molecular dynamics simulation of muscle versus TgACTI filaments confirms that much weaker lateral interactions are formed between protofilaments ( Fig. 4d ), consistent with previously identified residues that affect lateral contacts and filament stability [11] ( Fig. 4c ). 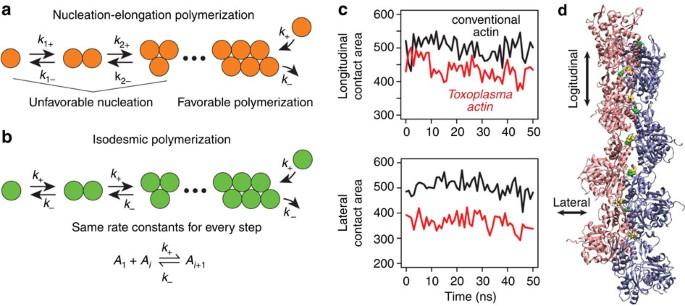Figure 4: Modeling filament polymerization and dynamics. (a,b) Standard nucleation–elongation mechanism versus isodesmic model. Under isodesmic polymerization, the on-rate (k+) and off-rate (k−) are the same for every monomer addition, independent of length. (c) Molecular dynamics simulation reflects a propensity for weaker lateral interactions inToxoplasmaversus muscle actin filaments (conventional). (d) Key amino-acid differences that were predicted to alter the lateral interaction between protofilaments11are highlighted in yellow and green, whereas the two strands of the filament are coloured blue and pink. Figure 4: Modeling filament polymerization and dynamics. ( a , b ) Standard nucleation–elongation mechanism versus isodesmic model. Under isodesmic polymerization, the on-rate ( k + ) and off-rate ( k − ) are the same for every monomer addition, independent of length. ( c ) Molecular dynamics simulation reflects a propensity for weaker lateral interactions in Toxoplasma versus muscle actin filaments (conventional). ( d ) Key amino-acid differences that were predicted to alter the lateral interaction between protofilaments [11] are highlighted in yellow and green, whereas the two strands of the filament are coloured blue and pink. Full size image Although this simple isodesmic model predicts the polymerization behaviour of TgACTI, across a range of concentrations, it does not address the depolymerization behaviour of filaments once they form. To examine this directly, we polymerized TgACTI at 20 μM in F-buffer overnight, then diluted it by fourfold, a concentration below the threshold where most of the actins form polymers of sufficient mass to sediment at 100,000 g ( Fig. 3a ). We observed a very gradual but significant decline in light scattering after dilution, which supports the conclusion that polymers of TgACTI have a slow off-rate. Again, the isodesmic model accurately fits the observations ( Fig. 3f ) but as there is no Cc, dilution results in loss of >30% of the polymer. In contrast, when ScACT filaments were diluted under similar conditions, they underwent more modest depolymerization and reached a new steady state where the free monomer concentration again equalled the Cc ( Fig. 3f ). ScACT depolymerization was accurately described by a nucleation–elongation model ( Fig. 3f ), which predicts only minor loss of polymer (that is, ~5%). Collectively, these observations fit the expectation that conventional actins are robust to depolymerization because they are naturally buffered by their Cc, whereas TgACTI respond more dramatically to alterations in concentration, thus resulting in filaments that are less stable. Collectively, our findings reveal that TgACTI slowly polymerizes to form a heterogeneous mixture of relatively short filaments, resulting in a length distribution remarkably different from that of conventional actins. This discovery explains previous differences from conventional actins and offers insight into the behaviour of parasite actin in vivo. First, nucleation is not rate limiting, so that T. gondii does not need nucleation-promoting factors. Indeed, homologues of actin-nucleating proteins, such as Arp2/3 complex, have not been identified within apicomplexan genomes [23] . Second, an isodesmic mechanism results in a distribution of small oligomers, which explains why TgACTI only sediments efficiently at higher g force [6] , [24] . Our findings also explain why long TgACTI filaments have not been observed in parasites by any method, including EM, fluorescence imaging of GFP–TgACTI and Ph staining [6] , [8] , [11] , [24] . Other parasite actin-binding proteins are also adapted to this difference in kinetics; for example, actin-depolymerizing factor (ADF) acts primarily as a sequestering agent while exhibiting minimal severing activity [25] , which is consistent with absence of stable filaments. As predicted by an isodesmic model, EM showed a distribution of heterogeneously sized small oligomers and short filaments ranging in size from 25 to 100 nm in length ( Fig. 1e , excluding bundles that may form by annealing of individual filaments). This size distribution is similar to filaments that form in vivo during gliding motility ( Fig. 1e and ref. 8 ). Previous studies have also shown that T. gondii has a streamlined repertoire of actin-binding proteins including ADF and profilin [25] , [26] . The ADF of T. gondii is somewhat unusual in functioning largely in sequestration of G-actin; the concentration of G-actin is ~35 μM in the cytosol, whereas that of TgACTI is ~40 μM (ref. 25 ). Combined with the affinity of TgADF for TgACTI (that is, 0.8 μM), it is likely that the majority of TgADF is bound to TgACTI [25] . In this regard, profilin has also been shown to function in sequestering TgACTI (~38 μM cytosolic concentration and a dissociation binding constant of ~5 μM) (ref. 26 ). Collectively, ADF and profilin should then combine to keep the concentration of free TgACTI monomer very low (that is, below 5 μM), a level that would only allow for the filaments to be short and of variable length. The robust control of free TgACTI levels, and hence the distribution of filament lengths, would appear to be of critical importance based on the observation that disruption of the genes encoding TgADF [27] or profilin [28] leads to profound defects in cell motility and cell invasion. Hence, isodesmic polymerization is better suited than nucleation–condensation for the assembly of short filaments and oligomers, which function in parasite motility rather than the long, stable filaments that represent the functioning form of F-actin in yeast and mammalian cells. Importantly, the fact that TgACTI undergoes isodesmic assembly does not make any a priori predictions about the directionality of assembly or the structure of the filament. Directionality during filament growth is determined by the on- and off-rate constants at the two ends of the filament, which are not required to be the same in an isodesmic process. Likewise, the net rate of assembly/disassembly may differ at the two ends, although such a difference would require energy, probably provided by ATP hydrolysis as is true for actins in general [29] . Determining the directionality of assembly is an important future goal that awaits methods for single-molecule imaging of TgACTI polymerization. An isodesmic polymerization process also does not imply that the structure of the TgACTI filament includes only a single protofilament. The reactions from monomer to dimer, dimer to trimer and so forth must have similar binding constants. The structural basis of this biochemical process is an open question that will require atomic-level structural and mutational analysis for proper resolution. At this point, we know that TgACTI filaments viewed by EM appear to display two protofilaments; however, the resolution was not sufficient to reveal whether the protofilaments are in a helical conformation. The filament may be in a relaxed conformation because of an intrinsically lower contribution of intra-strand interactions to filament stability, consistent with previous reports showing that TgACTI contains natural substitutions in residues that normally stabilize lateral interactions between the two protofilaments [11] . Thus, the subunit interactions that dominate during filament assembly may be arranged in a one-start helix. Bacterial actin-like proteins also form a variety of filament types ranging from single-strand protofilaments (that is, MreB) to both right- and left-handed helices comprising two protofilaments [17] . Collectively, these findings indicate that actin can adopt a wider range of conformations and assembly processes than those reflected by conventional actins in animal cells. Actin and related proteins have evolved to form higher order assemblies that perform mechanical work and impart structural rigidity [12] . Conventional eukaryotic actins use cooperative assembly to generate filaments with strong inter-strand contacts [30] . Prokaryotic actins such as the bacterial actin homologue MreB form both single-stranded helices and linear double-stranded filaments [31] , [32] , yet polymerization occurs by a nucleation–elongation mechanism with a Cc of ~0.9 μM (ref. 33 ). In contrast, TgACTI represents a different evolutionary strategy, utilizing an isodesmic process to form a double-stranded filament that lacks a cooperative mechanism of assembly and features weak inter-strand filament interactions. Our findings predict that other unconventional actins may also undergo a similar process of isodesmic polymerization. For example, Plasmodium ACTI shares many of the properties of TgACTI [11] , as do actins in many plants [34] , [35] and protozoan parasites [36] , [37] , [38] . In all these cases, actins exhibit unusual polymerization kinetics and remain primarily unpolymerized in vivo . Collectively, these observations are consistent with actin having adapted different modes of polymerization to support a diverse array of structural and motile processes in cells. Actin expression and purification TgACTI or ScACT were expressed and purified from baculovirus, as described previously [11] . In brief, His-tagged actins were purified using Ni–NTA agarose (Invitrogen) and stored in G-actin buffer (5 mM Tris-Cl, pH 8.0, 0.2 mM CaCl 2 , 0.2 mM ATP) containing 0.5 mM dithiothreitol with 100 μM sucrose. Purified actins were quantified as described [11] , stored at 4 °C and used within 2–3 days. Before use, purified actins were clarified by centrifugation at 100,000 g , 4 °C, for 30 min using a TL100 rotor and a Beckman Optima TL ultracentrifuge (Beckman Coulter, Brea, CA, USA). Polymerization properties of actins diluted in G-buffer were examined following addition of F-buffer (final: 50 mM KCl, 2 mM MgCl 2 , 1 mM ATP, 1 mM EGTA at pH 8.0) or in KMEI (final: 50 mM KCl, 10 mM imidazole, 2 mM MgCl 2 , 1 mM EGTA, pH 7.2). Light scattering Actins were diluted in G-buffer, and polymerization was induced by addition of F-buffer (pH 8.0; with 1 mM EGTA to replace bound Ca 2+ with Mg 2 ). Ninety-degree light scattering was monitored in a 100-μl cuvette (Submicro Quartz Fluorometer cell, Starna Cells, Atascadero, CA, USA) using a PTI Quantmaster spectrofluorometer (Photon Technology International, Santa Clara, CA, USA): excitation 310 nm (1 nm bandpass), emission 310 nm (1 nm bandpass), as described previously [11] . Data were collected either during the first 100 min to capture initial kinetics or after 20 h to establish the steady-state level of polymerization (as established by testing different time intervals). The average reading at 20 h was plotted versus protein concentrations and analysed using linear and non-linear functions (Prism, GraphPad). To properly normalize the depolymerization data, we rescaled the data based on knowledge of the expected starting and ending F-actin concentrations based on sedimentation experiments. Polymerization model To describe the polymerization kinetics, we adopted an isodesmic polymerization model. This model assumes that the association and dissociation rate constants are identical for all steps of the polymerization reaction. We explicitly modelled each polymer length by solving the coupled set of differential equations for the set of reactions keeping track of all polymers up to a length of i =100 protomers. The amount of polymer was simply taken as the sum of all oligomers (dimers, trimers and so on), and this quantity was used for comparison with both light scatting and sedimentation data. The set of rate constants that gave us the best least-squares fits to the polymerization and depolymerization data were k on =5.9 × 10 −5 μM −1 s −1 and k off =4.0 × 10 −4 s −1 . Molecular dynamics simulations We used the results of molecular dynamics simulations described previously [11] . The pairwise contact surface area was calculated and averaged over all protomers using Visual Molecular Dynamics (VMD) [39] . Fluorescence microscopy Purified recombinant actins were diluted in F-buffer (pH 8.0)±equimolar unlabelled Ph (Molecular Probes, Eugene, OR, USA) and Alexa-488 phalloidin (0.33 μM; Molecular Probes), incubated for 1 h and viewed with a Zeiss Axioskop (Carl Zeiss, Thornwood, NY, USA) using 63X Plan-NeoFluar oil immersion lens (1.30 NA). Images were collected using a Zeiss Axiocam with Axiovision v3.1 and processed by linear adjustment using Photoshop v8.0 (Adobe, San Jose, CA, USA). Electron microscopy Purified recombinant TgACTI and ScACT were diluted to 40 and 5 μM, respectively, in F-buffer and polymerized for 1 h. Quick-freeze, deep-etch EM of samples on mica was performed as described previously [40] . Replicas were mounted on formvar-coated copper grids and photographed with a JEOL 1400 microscope (Tokyo, Japan) with an AMT digital camera (Woburn, MA, USA). Actin sedimentation assays Purified recombinant actins were diluted in G-buffer and then incubated in F-buffer (pH 8.0) or KMEI (pH 7.2) for 1 h at room temperature and centrifuged at 100,000 g using a TL100 rotor and Beckman Optima TL ultracentrifuge. To examine the effects of Ph on polymerization, samples were incubated in F-buffer (pH 8.0)±equimolar unlabelled Ph (Molecular Probes) for 1 h at room temperature and centrifuged at 100,000 or 350,000 g for 1 h at room temperature. Acetone-precipitated supernatants and pellets were resolved on a 12% SDS–PAGE gels, stained with Sypro-Ruby (Molecular Probes), visualized using an FLA-5000 phosphorimager (Fuji Film Medical Systems) and quantified using Image Gauge v4.23. To establish the extent of polymerization at steady state, samples were polymerized in F-buffer (pH 8.0) for 20 h at room temperature and sedimented at 100,000 g . The ratio of the pellet/total actin at 20 h was plotted using a sigmoidal dose response (Prism, GraphPad). Density centrifugation Purified recombinant actins were incubated with 1 mM EGTA and 50 μM MgCl 2 for 10 min (to replace bound Ca 2+ with Mg 2+ ). Actins were incubated in G-buffer, F-buffer (pH 8.0) or F-buffer supplemented with equimolar Ph (Molecular Probes) for 1 h at room temperature. Samples were loaded on the top of 11 ml 5–40% continuous sucrose gradients, made in the corresponding buffer using an Auto Densi-Flow Gradient Fractionator (LabConco, Kansas City, MO, USA) and centrifuged at 100,000 g , 4 °C for 20 h using a SW41 rotor in an L-80 ultracentrifuge (Beckman Coulter). BSA, 4.4S, lactate dehydrogenase, 7S, catalase, 11.4S, thyroglobulin, 19.4S (HMW Calibration kit, GE Healthcare, Buckinghamshire, UK) were used for density standards. The specific gravity of each fraction was measured using a refractometer (Sper Scientific, Scottsdale, AZ, USA). Fractions were precipitated in 10% trichloroacetic acid for 1 h, resolved on 12% SDS–polyacrylamide gels, stained with Sypro-Ruby (Molecular Probes), visualized using an FLA-5000 phosphorimager (Fuji Film Medical Systems) and Image Gauge v4.23. Dynamic light scattering Purified recombinant TgACTI and ScACT were clarified as described above and diluted to either 1 or 5 μM in G-buffer or to 1 or 5 μM in F-buffer (pH 8.0) and polymerized for 1 h. Dynamic light scattering was performed using DynaPro-MSXTC (Wyatt Technology, Santa Barbara, CA, USA) and analysed using Dynamics V6.3.4.0 software (Wyatt Technology). Circular dichroism Purified recombinant actins were diluted to 0.4 μM in 0.8 M sodium fluoride buffer and loaded into a 10-mm cuvette for measurement. Circular dichroism spectra were monitored at 200–250 nm using a Jasco J-810 Spectrometer (Jasco Analytical Instruments, Easton, MD, USA). Data were plotted using Prism (GraphPad). Estimation of hydrodynamic radii To estimate the hydrodynamic radii of different-sized actin oligomers, we used the Oda et al. [30] actin filament structure and created structures for the monomer, low-pitch and high-pitch dimers, trimers and so on. Using HYDROPRO [41] , we calculated the translational diffusion contact at 20 °C and used this value to determine the corresponding Rh based on Stokes–Einstein theory. How to cite this article: Skillman, K. M. et al. The unusual dynamics of parasite actin result from isodesmic polymerization. Nat. Commun. 4:2285 doi: 10.1038/ncomms3285 (2013).